The earliest known stem-tetrapod from the Lower Devonian of China Recent discoveries of advanced fish-like stem-tetrapods (for example, Panderichthys and Tiktaalik ) have greatly improved our knowledge of the fin-to-limb transition. However, a paucity of fossil data from primitive finned tetrapods prevents profound understanding of the acquisition sequence of tetrapod characters. Here we report a new stem-tetrapod ( Tungsenia paradoxa gen. et sp. nov.) from the Lower Devonian (Pragian, ∼ 409 million years ago) of China, which extends the earliest record of tetrapods by some 10 million years. Sharing many primitive features with stem-lungfishes, the new taxon further fills in the morphological gap between tetrapods and lungfishes. The X-ray tomography study of the skull depicts the plesiomorphic condition of the brain in the tetrapods. The enlargement of the cerebral hemispheres and the possible presence of the pars tuberalis in this stem-tetrapod indicate that some important brain modifications related to terrestrial life had occurred at the beginning of the tetrapod evolution, much earlier than previously thought. Living tetrapods, such as the frogs, turtles, birds and mammals, are a subgroup of the tetrapod lineage (tetrapod total group or tetrapodomorphs). The lineage also includes finned and limbed tetrapods that are more closely related to living tetrapods than to living lungfishes [1] , [2] , [3] . Previously, the undisputed earliest known stem-tetrapod was Kenichthys , a finned member from the late Emsian ( ∼ 399 million years ago (mya)) of Yunnan, China [4] , [5] . By comparison, the oldest fossil record of the lungfish lineage (dipnomorphs), which forms the immediate sister group of tetrapodomorphs, can be traced back to the early Lochkovian ( ∼ 415 mya) [6] . Thus, a ghost lineage of at least 16 million years existed for the tetrapod total group [7] , [8] . Here, we describe a new finned stem-tetrapod, Tungsenia paradoxa gen. et sp. nov., from the Lower Devonian (Pragian, ∼ 409 mya) of Yunnan, China. The new taxon is ∼ 10 million years older than Kenichthys , and shifts the beginning of stem-tetrapods back to the Pragian. The parietal shield (holotype, V10687) and two lower jaws (V10688.1-2) were originally described as an indeterminate osteolepid [9] . However, these specimens were not fully prepared and their phylogenetic position was open to question. After the discovery of complementary specimens (V15132.1-22) from the same locality, we further prepared the original material to unveil the medial aspect of mandible and hitherto unrecognised aspects of the neurocranial anatomy. Geological setting The new material was recovered from a yellow sandstone layer of the Posongchong Formation, near the dam of the Qingmen Reservoir in the suburb of Zhaotong, northeastern Yunnan, South China ( Fig. 1 ). The Posongchong fauna includes diverse galeaspid agnathans [9] , [10] , [11] , [12] , placoderms [13] , [14] , onychodonts, coelacanths and rhipidistians [9] , [15] , [16] , [17] , [18] ( Supplementary Table S1 ), as well as lingulids and plant remains [15] , [19] . 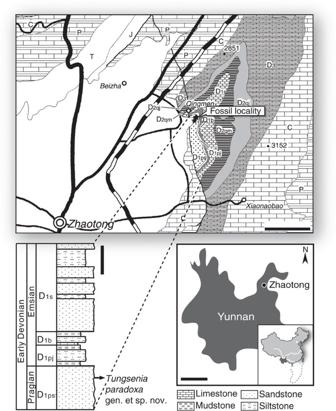Figure 1: Location map and lithocolumn ofTungsenia paradoxagen. et sp. nov. C, Carboniferous; D1b, Bianqinggou Formation; D1pj, Pojiao Formation; D1ps, Posongchong Formation; D1s, Suotoushan Formation; D2qj, Qujing Formation; D2qm, Qingmen Formation; D3, Zaige Formation; J, Jurassic; P, Permian; T, Triassic. Scale bar, above, 3 km; below left, 100 m; below right, 100 km. Figure 1: Location map and lithocolumn of Tungsenia paradoxa gen. et sp. nov. C, Carboniferous; D1b, Bianqinggou Formation; D1pj, Pojiao Formation; D1ps, Posongchong Formation; D1s, Suotoushan Formation; D2qj, Qujing Formation; D2qm, Qingmen Formation; D3, Zaige Formation; J, Jurassic; P, Permian; T, Triassic. Scale bar, above, 3 km; below left, 100 m; below right, 100 km. Full size image This clastic fish-bearing stratum was originally named as the ‘Cuifengshan Formation’, by comparsion to the Cuifengshan Group (previously the Cuifengshan Formation) in neighbouring Qujing district, Yunnan [20] , [21] . However, considering the lithology and faunal composition, as well as the overlying strata, the Devonian sediments underlying the marine Pojiao Formation in Zhaotong are more suggestive of the Posongchong Formation in Wenshan and Guannan, southeastern Yunnan than the Cuifengshan Group in Qujing. In this regard, the Posongchong Formation was proposed to represent the lowermost formation of the Devonian sequence in Zhaotong [9] , [15] , [16] , [17] , [18] , [19] . Systematic palaeontology Osteichthyes Huxley, 1880 Sarcopterygii Romer, 1955 Tetrapodomorpha Ahlberg, 1991 Tungsenia gen. nov. Etymology. Generic name after Liu Tungsen for his pio neering contribution to Paleoichthyology in China. Type species. T. paradoxa sp. nov. Diagnosis. A small cosmine-covered stem-tetrapod char acterized by having a large orbital notch ∼ 40% of total parietal shield length, pineal foramen at the middle level of orbits, a large pair of fangs on the parasymphysial plate, short robust olfactory tracts, developed cerebral cavity, pineal and parapineal recesses not extending anteriorly, hypophysial fossa far posterior to the optic nerve root and paired tongue-like recesses at the front of the hypophysial fossa. Tungsenia paradoxa sp. nov. Etymology. Specific name from the Latin paradoxus , unexpected. Holotype. IVPP V10687, a parietal shield. Referred material. Skulls, V15132.1-6; lower jaws,  V10688.1-2, V15132.7-20; cheek bone, V15132.22. Type locality. Zhaotong, Yunnan Province, China. Formation and age. Posongchong Formation (Pragian, Early Devonian). Diagnosis. As for the generic diagnosis. Description The parietal shield is about as wide as it is long ( Fig. 2 ). In profile, the shield presents a protruding and slightly upturned snout, suggesting that the mouth was subterminal. The orbital notch, comprising ∼ 40% of total parietal shield length, is the largest among that of stem-tetrapods. The pineal foramen is anteriorly positioned, corresponding to the midpoint of the orbits. 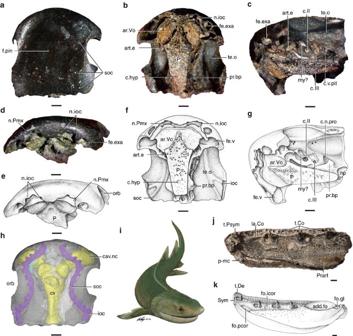Figure 2:Tungsenia paradoxagen. et sp. nov. from the Lower Devonian of China. Holotype (IVPP V10687), parietal shield in dorsal (a), ventral (b, photo;f, line drawing), ventrolateral (c, photo;g, line drawing) and anterior (d, photo;e, line drawing) views, and its rendered translucent showing endocranial cavity in dorsal view (h). (i) Restoration of external morphology. (j) Right mandible (IVPP V15132.7) in mesial view. (k) Restoration of mandible in mesial view. add.fo, adductor fossa; art.e, ethmoid articulation; ar.Vo, vomeral area; cav.nc, cavity of nasal capsule; c.hyp, canal for buccohypophysial duct; c.n.pro, canal for profundus branch of trigeminal nerve; cv, cranial cavity; c.v.pit, canal for pituitary vein; c.II, canal for optic nerve; c.III, canal for oculomotor nerve; fe.exa, fenestra exonarina anterior; fe.v, fenestra ventralis; fo.gl, glenoid fossa; fo.icor, intercoronoid fossa; fo.pcor, precoronoid fossa; f.pin, pineal foramen; ioc, infraorbital canal; la.Co, tooth pavement on the lateral portion of coronoids; my?, myodome for eye muscle attachment?; n.ioc, notch for infraorbital canal; n.Pmx, notch for premaxillary; np, notochordal pit; orb, orbital notch; P, parasphenoid; p-mc, pores for mandibular canal; Prart, prearticular; pr.bp, basipterygoid process; soc, supraorbital canal; Sym, symphysial area; t.Co, coronoid tusks; t.De, dentary teeth; te.o, orbital tectum; t.Psym, parasymphysial plate tusk. Scale bar, 1 mm. Figure 2: Tungsenia paradoxa gen. et sp. nov. from the Lower Devonian of China. Holotype (IVPP V10687), parietal shield in dorsal ( a ), ventral ( b , photo; f , line drawing), ventrolateral ( c , photo; g , line drawing) and anterior ( d , photo; e , line drawing) views, and its rendered translucent showing endocranial cavity in dorsal view ( h ). ( i ) Restoration of external morphology. ( j ) Right mandible (IVPP V15132.7) in mesial view. ( k ) Restoration of mandible in mesial view. add.fo, adductor fossa; art.e, ethmoid articulation; ar.Vo, vomeral area; cav.nc, cavity of nasal capsule; c.hyp, canal for buccohypophysial duct; c.n.pro, canal for profundus branch of trigeminal nerve; cv, cranial cavity; c.v.pit, canal for pituitary vein; c.II, canal for optic nerve; c.III, canal for oculomotor nerve; fe.exa, fenestra exonarina anterior; fe.v, fenestra ventralis; fo.gl, glenoid fossa; fo.icor, intercoronoid fossa; fo.pcor, precoronoid fossa; f.pin, pineal foramen; ioc, infraorbital canal; la.Co, tooth pavement on the lateral portion of coronoids; my?, myodome for eye muscle attachment? ; n.ioc, notch for infraorbital canal; n.Pmx, notch for premaxillary; np, notochordal pit; orb, orbital notch; P, parasphenoid; p-mc, pores for mandibular canal; Prart, prearticular; pr.bp, basipterygoid process; soc, supraorbital canal; Sym, symphysial area; t.Co, coronoid tusks; t.De, dentary teeth; te.o, orbital tectum; t.Psym, parasymphysial plate tusk. Scale bar, 1 mm. Full size image Tungsenia resembles Kenichthys [4] , [5] and basal dipnomorphs (for example, Youngolepis and Powichthys ) [22] , [23] , [24] in the medioventrally directed snout, the infraorbital sensory canal running along the suture between the premaxillary and neighbouring bones, the broad orbital tectum and the well-developed basipterygoid processes ( Fig. 2a–g ). The elongated, broad parasphenoid and the paired internasal pits ( Fig. 2b ; Supplementary Fig. S3b ) are shared with primitive sarcopterygian Styloichthys and basal dipnomorphs [8] , [22] , [24] , [25] , but differing from the remainder of the stem-tetrapods [4] , [26] , [27] , [28] ( Supplementary Fig. S4 ). A teardrop-shaped recess ( Fig. 2c ) is located anterodorsal to the optic foramen. A similar recess is also found in many finned stem-tetrapods, such as Gogonasus , Medoevia , Cladarosymblema and Litoptychus , and has been interpreted as the attachment area for eye muscle [26] , [28] , [29] , [30] , [31] . Other features shared with stem-tetrapods include the opening for the pituitary vein at the base of the basipterygoid process and a flat parasymphysial dental plate [1] , [30] . A large pair of fangs on the parasymphysial plate ( Fig. 2j ; Supplementary Fig. S3c,e ) is comparable to that in limbed stem-tetrapods (for example, Ichthyostega and Acanthostega ) [32] , but absent in finned stem-tetrapods, suggesting that the parasymphysial fang pair has evolved in parallel within the tetrapod lineage. A compound cheek plate, comprising a fused squamosal+quadratojugal+preopercular ( Fig. 3a ), is similar to that in the dipnomorph Youngolepis and some finned stem-tetrapods ( Supplementary Fig. S5a–c ) [33] , [34] , [35] . As inferred from the anterior overlap area on the cheek plate, the postorbital bone was proportionally large as in the rhizodont Barameda [36] ( Supplementary Fig. S5d ). 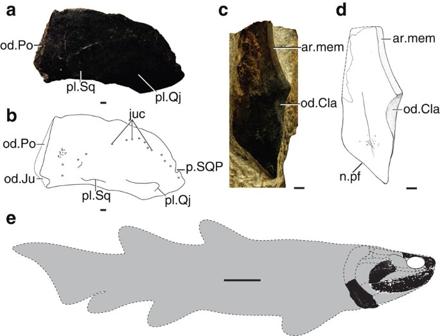Figure 3: Tungsenia paradoxa gen. et sp. nov. Compound cheek bone (Sq+Qj+Pop) (V15132.22) in external view (a, photo;b, line drawing). Left cleithrum in external view (c, photo;d, line drawing). (e) Tentative reconstruction based on available materials (in black). ar.mem, area for attachment of membraneous posterior wall of branchial cavity; juc, jugal canal; n.pf, notch for peoral fin; od.Cla, overlap area for clavicle; od.Ju, overlap area for jugal; od.Po, overlap area for postorbital; p.SQP, external pit on Sq+Qj+Pop; pl.Qj, quadratojugal pit-line; pl.Sq, squamosal pit-line. Scale bar, above, 1 mm; below, 1 cm. Figure 3: Tungsenia paradoxa gen. et sp. nov. Compound cheek bone (Sq+Qj+Pop) (V15132.22) in external view ( a , photo; b , line drawing). Left cleithrum in external view ( c , photo; d , line drawing). ( e ) Tentative reconstruction based on available materials (in black). ar.mem, area for attachment of membraneous posterior wall of branchial cavity; juc, jugal canal; n.pf, notch for peoral fin; od.Cla, overlap area for clavicle; od.Ju, overlap area for jugal; od.Po, overlap area for postorbital; p.SQP, external pit on Sq+Qj+Pop; pl.Qj, quadratojugal pit-line; pl.Sq, squamosal pit-line. Scale bar, above, 1 mm; below, 1 cm. Full size image A reconstruction of the skull and endocast based on high-resolution computed tomography (HRCT) ( Figs 2h and 4 ; Supplementary Movies 1 and 2 ) reveals an unexpected combination of brain features seen in Tungsenia . The short olfactory tracts and the anteriorly extending brain cavity recall the conditions in fossil sharks and placoderms [37] , [38] ( Supplementary Fig. S9 ). Besides, the brain and nerves exhibit a previously unrecognized mosaic of tetrapod and lungfish traits. The olfactory tracts of Tungsenia resemble those of basal dipnomorphs (for example, Porolepis and Glyptolepis ) [25] in anteriorly diverging with an angle up to 60°. Posteriorly, the space for the hemispheres (cerebral cavity) is swollen and enlarged, comparable to that in many other stem-tetrapods [27] , [39] . Although the enlargement of the hemispheres has independently evolved among different major groups such as cartilaginous fishes and ray-finned fishes, the evidence from Tungsenia suggests that the enlarged hemispheres in the tetrapodomorphs appeared during the incipient stage of their evolution ( Fig. 5 ). 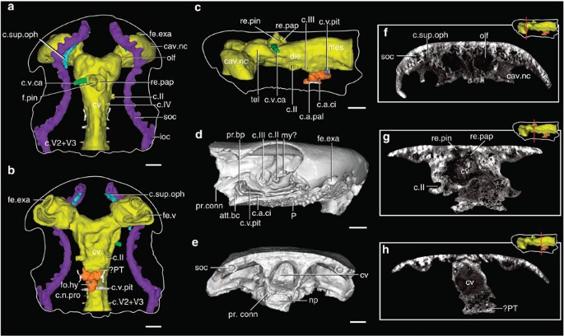Figure 4: Digital restorations ofTungsenia paradoxagen. et sp. nov. (a–c) Digital endocasts of dorsal (a), ventral (b) and left lateral (c) views. (d,e) Braincase in right lateral (d) and posterior (e) views. Selected transverse CT scan slices through the endocranial cavity, showing the brain cavity at the level of the olfactory tract (f), the opening for pineal organ (g) and the anterior part of the hypophysial fossa (h) att.bc, attachment for basicranial muscle; c.a.ci, canal for internal carotid artery; c.a.pal, canal for palatine artery; c.sup.oph, canal for superficial ophthalmic nerve; c.v.ca, canal for anterior cerebral vein; c.IV, canal for trochlear nerve; c.V2+V3, canal for maxillary and mandibular branch of trigeminal nerve; die, diencephalon; fo.hy, hypophysial fossa; mes, mesencephalon; olf, olfactory tract; pr.conn, processus connectens; re.pap, recess for parapineal organ; re.pin, recess for pineal organ; tel, telencephalon; ?PT, paired tongue-like recesses at the front of the hypophysial fossa, possibly housing the pars tuberalis. For other abbreviations seeFig. 2. Scale bar, 1 mm. Figure 4: Digital restorations of Tungsenia paradoxa gen. et sp. nov. ( a – c ) Digital endocasts of dorsal ( a ), ventral ( b ) and left lateral ( c ) views. ( d , e ) Braincase in right lateral ( d ) and posterior ( e ) views. Selected transverse CT scan slices through the endocranial cavity, showing the brain cavity at the level of the olfactory tract ( f ), the opening for pineal organ ( g ) and the anterior part of the hypophysial fossa ( h ) att.bc, attachment for basicranial muscle; c.a.ci, canal for internal carotid artery; c.a.pal, canal for palatine artery; c.sup.oph, canal for superficial ophthalmic nerve; c.v.ca, canal for anterior cerebral vein; c.IV, canal for trochlear nerve; c.V2+V3, canal for maxillary and mandibular branch of trigeminal nerve; die, diencephalon; fo.hy, hypophysial fossa; mes, mesencephalon; olf, olfactory tract; pr.conn, processus connectens; re.pap, recess for parapineal organ; re.pin, recess for pineal organ; tel, telencephalon; ?PT, paired tongue-like recesses at the front of the hypophysial fossa, possibly housing the pars tuberalis. For other abbreviations see Fig. 2 . Scale bar, 1 mm. 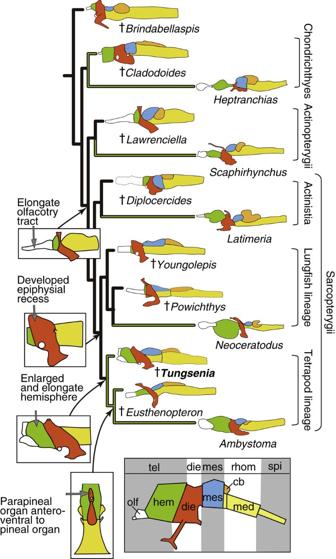Figure 5: Patterns of brain evolution in selected jawed vertebrates. The brains (extant taxa) or endocasts (extinct taxa) are shown in lateral views. The bold green lines indicate that the enlarged hemispheres have independently evolved several times among different groups. The enlarged hemispheres had occurred at the initial stage of the tetrapod evolution.†represents extinct taxa. The vertebrate brain archetype is modified after Striedter44and the brains of living taxa are modified after Nieuwenhuys45. cb, cerebellum; hem, hemisphere; med, medulla; rhom, rhombencephalon; spi, spinal cord. For other abbreviations seeFig. 4. Not to scale. Full size image Figure 5: Patterns of brain evolution in selected jawed vertebrates. The brains (extant taxa) or endocasts (extinct taxa) are shown in lateral views. The bold green lines indicate that the enlarged hemispheres have independently evolved several times among different groups. The enlarged hemispheres had occurred at the initial stage of the tetrapod evolution. † represents extinct taxa. The vertebrate brain archetype is modified after Striedter [44] and the brains of living taxa are modified after Nieuwenhuys [45] . cb, cerebellum; hem, hemisphere; med, medulla; rhom, rhombencephalon; spi, spinal cord. For other abbreviations see Fig. 4 . Not to scale. Full size image Immediately behind the cerebral cavity, the neuro-epiphysial recess presents laterally adjacent pineal and parapineal organs ( Fig. 4a ) as in basal dipnomorphs [25] , [40] . However, unlike other rhipidistians (the lungfish plus tetrapod lineages) [41] , these two organs do not extend forward or form canal-like structures. The mesencephalic portion is more than half of the length of the cranial cavity, which recalls the condition in placoderms [38] . Laterally, both trigeminal and profundus nerves emerge through foramina in the ethmosphenoid ( Fig. 4a ), like those of Youngolepis and Powichthys [22] , [40] . The hypophysial fossa ( Fig. 4b ), as in Youngolepis and Powichthys , is stout and triangular. However, the fossa is placed in a far more posterior position relative to the optic nerve root. A pair of tongue-like recesses at the front of the hypophysial fossa ( Fig. 4b ) may topologically correspond to the paired neurocranial structures housing the pars tuberalis (PT) in living urodeles ( Supplementary Fig. S8 ). Incidentally, a paired tube-like structure at the front of the hypophysial fossa in the dipnomorph Glyptolepis was identified as the ‘pars tuberalis’ (PT) [25] , [27] . However, it differs from the condition in Tungsenia and living urodeles in connecting directly with the brain cavity [25] , and additional investigation of the ‘PT’ of Glyptolepis is required. The distal part of the hypophysial fossa of Tungsenia is connected with a complex of parallel canals for blood vessels, as in Youngolepis and Powichthys [22] , [40] . The hypophysial canal is funnel-shaped, extending posteriorly to set its opening on the parasphenoid far from the optic nerve exit ( Fig. 4c ; Supplementary Fig. S8a,b ). A phylogenetic analysis of 38 taxa, including 21 stem-tetrapods, shows that Tungsenia is at the most basal position of the tetrapod stem lineage ( Fig. 6 ; Supplementary Figs S1 and S2 ). At least two unambiguous synapomorphies demonstrate the stem-tetrapod affinity of Tungsenia : the pituitary vein opening anteroventral to the basipterygoid process, and the flat parasymphysial plate of mandible. 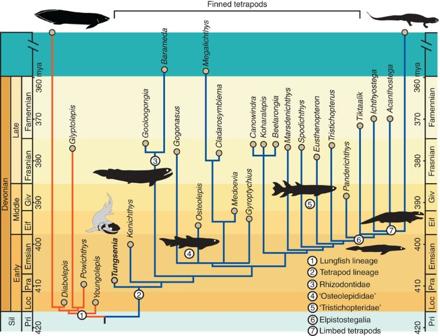Figure 6: Temporally calibrated cladogram of the simplified strict consensus tree. Tungsenia, the basalmost member of the stem-tetrapods (seeSupplementary Methods), extends the fossil record of the tetrapod lineage by 10 million years. The first diversification of limbed tetrapods is positioned before the early Middle Devonian, based on the limbed tetrapod trackways from Poland46. The lungfish lineage is in orange. Figure 6: Temporally calibrated cladogram of the simplified strict consensus tree. Tungsenia , the basalmost member of the stem-tetrapods (see Supplementary Methods ), extends the fossil record of the tetrapod lineage by 10 million years. The first diversification of limbed tetrapods is positioned before the early Middle Devonian, based on the limbed tetrapod trackways from Poland [46] . The lungfish lineage is in orange. Full size image The basal phylogenetic position, unique character combination and earlier occurrence of Tungsenia have wide implications for the study of the tetrapod ancestry. First, Tungsenia pushes back the fossil record of tetrapods by some 10 million years into the Pragian. As a result, the first appearance of the tetrapod total group has now been drawn far closer to the estimated time of the lungfish–tetrapod split [7] . Second, Tungsenia displays a mixture of endocranial features previously found either in basal dipnomorphs (for example, paired internasal pits, broad parasphenoid and exits for trigeminal and profundus nerves in the parietal shield) or in tetrapodomorphs (for example, the position of the pituitary vein opening). It further fills in the morphological gap between tetrapods and lungfishes, and unveils the evolutionary pattern of character changes during the initial diversification of stem-tetrapods. Different from the mosaic cranial features, the mandible of Tungsenia displays undisputed stem-tetrapod features, suggesting that, at the early stage of the tetrapod evolution, changes in mandible were faster than changes in endocranium. Last, the HRCT study of Tungsenia provides unique insights into the incipient stage of tetrapod brain evolution. For a long time, our knowledge of the brain evolution in stem-tetrapods was limited owing to a small selection of well-studied taxa [27] , [38] , [39] , [42] . Thus, the investigation of the brain in Tungsenia , the basalmost stem-tetrapod, is crucial for revealing the acquisition sequence of tetrapod brain features. The digital endocast of Tungsenia shows many plesiomorphies shared with stem-lungfishes and non-sarcopterygian taxa, such as placoderms and early sharks. Such arrangement indicates that the accelerated brain modifications (for example, developed olfactory bulbs, longitudinally positioned pineal and parapineal canals, and shorten mesencephalon) of stem-tetrapods had happened crownward of Tungsenia . On the other hand, the inferred enlarged hemispheres of Tungsenia indicate that the enlargement of the hemispheres had occurred at the beginning of the tetrapod evolution. In addition, although the homologous comparisons among the PT of living tetrapods, the ‘PT’ of Glyptolepis and the paired tongue-like recesses of Tungsenia still need additional investigations to test, the newly identified recesses in an early stem-tetrapod seem to provide a potential to recognize that the PT, a structure linked with some adaptation necessary for terrestrial living modes, had a deeper origin than previously considered. Phylogenetic analysis A phylogenetic analysis was performed on a matrix of 263 characters scored for 38 taxa (see Supplementary Methods ). All characters were treated as unordered, and weighted equally. The resulting data matrix was subjected to the parsimony analysis in PAUP* (version 4.0b10) [43] using a heuristic search, with Guiyu , Psarolepis and Achoania (basal osteichthyans) specified as the outgroup. The analysis generated five most parsimonious trees with 579 steps (Consistency index=0.5250; Homoplasy index=0.4750; Retention index=0.7255; and Rescaled consistency index=0.3809). All trees show Tungsenia as the most basal stem-tetrapod. The strict consensus tree ( Supplementary Fig. S1a ) highlights the poor phylogenetic resolution of the ‘Osteolepiformes’. X-ray micro-tomography HRCT data were acquired at the Australian National University in 2007. Spatial resolution was set to 11.9 μm, (1024) [3] 16-bit voxels, 80 kV and 60 mA. Slice data derived from the scans were then analysed and manipulated using Drishti software. The three-dimensional reconstructions were created in the Mimics (v13.1) software. The images of the reconstructions were exported from Mimics and VG Studio Max (v2.0), and finalized in Adobe Photoshop. Nomenclatural acts This published work and the nomenclatural acts it contains have been registered in ZooBank, the proposed online registration system for the International Code of Zoological Nomenclature (ICZN). The ZooBank LSIDs (Life Science Identifiers) can be resolved and the associated information viewed through any standard web browser by appending the LSID to the prefix ‘ http://zoobank.org/ ’. The LSID for this publication is: urn:lsid:zoobank.org:act:39677617-77C8-4144-800E-59C595E66DE8; urn:lsid:zoobank.org:pub:F80BD663-B04C-46E9-A245-1DCF0FB8383B. How to cite this article: Lu, J. et al. The earliest known stem-tetrapod from the Lower Devonian of China. Nat. Commun. 3:1160 doi: 10.1038/ncomms2170 (2012).